No specific relationship between hypnotic suggestibility and the rubber hand illusion 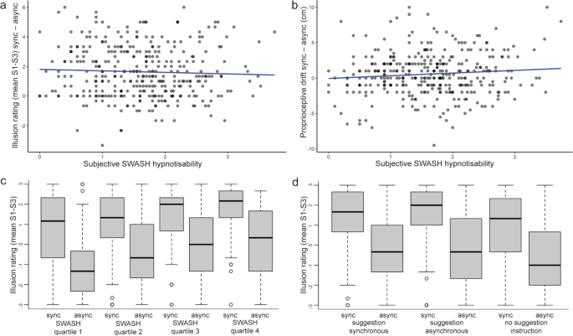Fig. 1: The rubber hand illusion (RHI) is resistant to hypnotic suggestibility. aNo significant relationship between trait hypnotic suggestibility (SWASH) and illusion ratings (mean of questionnaire statements S1 to S3) when comparing the synchronous (illusion) and asynchronous (control) conditions (ϱ = −0.066,p= 0.219, 95% CI [−0.169, 0.039], BF01= 5.685,n= 353).bSimilarly, there was no significant relationship between SWASH and proprioceptive drift when contrasting the conditions (ϱ = 0.047,p= 0.376, 95% CI [−0.057, 0.151], BF01= 1.657,n= 353).cWhen dividing the participants into four quartiles based on the trait of hypnotic suggestibility (SWASH quartiles 1–4), the illusion is significantly induced in all groups, including the least hypnotically suggestible subjects (quartile 1). The differences in illusion ratings between the synchronous and asynchronous conditions were significant in all four quartiles (1:V= 2575.5,p< 0.001,n= 88; 2:V= 2932,p< 0.001,n= 89; 3:V= 3198,p< 0.001,n= 92; 4:V= 2779.5,p< 0.001,n= 84), and the synchronous conditions were always rated significantly >0 (1:V= 2387.5,p< 0.001; 2:V= 3258.5,p< 0.001; 3:V= 3724,p< 0.001; 4:V= 3271.5,p< 0.001). Moreover, non-parametric one-way ANOVA (Kruskal–Wallis H test) on difference in illusion ratings between the synchronous and the asynchronous conditions in four quartiles was not significant (χ2 = 2.913, df = 3,p= 0.405; a direct comparison between quartile 1 and quartile 4 in terms of condition-specific differences was also non-significant:W= 3879.5,p= 0.574).dExplicit suggestions before the experiment commenced did not influence the illusion since the difference in illusion rating between the synchronous and asynchronous condition was not significantly different in the three groups that were informed that they would experience the strongest illusion in the synchronous condition (suggestion synchronous;n= 114), in the asynchronous condition (suggestion asynchronous;n= 115) or when receiving no information (no suggestion instruction;n= 124) (suggestion sync vs suggestion async:W= 6382,p= 0.73; suggestion sync vs no suggestion instruction:W= 7178,p= 0.836; suggestion async vs no suggestion instruction:W= 7422.5,p= 0.584). In all three groups, the illusion was significantly induced when contrasting the two conditions (V= 5438,p< 0.001;V= 4697,p< 0.001;V= 5169.5,p< 0.001). The data from Lush et al.1are openly available and were analyzed with RStudio software, version 1.3.1056, and the BayesFactor software package, version 0.9.12–4.2. Non-parametric tests were used (Wilcoxon signed-rank test for paired comparisons, Mann–WhitneyUtest for independent group comparisons) since the questionnaire data were ordinal and not normally distributed; two-tailed tests were performed. For the Bayes factor analysis, the default Cauchy priors were used. Sync synchronous condition, Async asynchronous condition, SWASH Sussex-Waterloo Scale of Hypnotizability. The boxplots (incandd) depict the data based on their median (thick black line) and quartiles (upper and lower ends of boxes). The vertical lines, i.e., the whiskers, indicate the minimum or maximum values within 1.5x the interquartile range above and below the upper and lower quartile. The circles denote outlier observations, the furthest being the minimum or maximum values in the data. Further information on research design is available in the Nature Research Reporting Summary linked to this article.